Strongly interacting confined quantum systems in one dimension In one dimension, the study of magnetism dates back to the dawn of quantum mechanics when Bethe solved the famous Heisenberg model that describes quantum behaviour in magnetic systems. In the last decade, one-dimensional (1D) systems have become a forefront area of research driven by the realization of the Tonks–Girardeau gas using cold atomic gases. Here we prove that 1D fermionic and bosonic systems with strong short-range interactions are solvable in arbitrary confining geometries by introducing a new energy-functional technique and obtaining the full spectrum of energies and eigenstates. As a first application, we calculate spatial correlations and show how both ferro- and antiferromagnetic states are present already for small system sizes that are prepared and studied in current experiments. Our work demonstrates the enormous potential for quantum manipulation of magnetic correlations at the microscopic scale. Strongly interacting quantum particles are ubiquitous in nature and play a vital role in superfluidity, superconductivity and magnetism, and low-dimensional magnetic systems have great potential to deliver the key insights into fundamental properties of the materials used in modern technology [1] . The study of magnetism in one-dimension (1D) goes back to the dawn of quantum mechanics when Bethe solved the Heisenberg model by introducing the famous Bethe ansatz method [2] . During the 1960s the technique was used to solve several paradigmatic models including the Lieb–Liniger model of repulsive bosons [3] , impurity problems with fermions by McGuire [4] , [5] and Yang’s solutions of homogeneous two-component Fermi systems [6] that led to Lieb and Wu’s solution of the 1D Hubbard model in 1968 (ref. 7 ). Common to the theoretical models is that periodic or open boundaries are essential ingredients, and the Bethe ansatz cannot be applied for general confinement, which is nevertheless the reality in many state-of-the-art set-ups that have for instance been used to realize the Tonks–Girardeau [8] , [9] gas using cold bosonic atoms [10] , [11] , [12] . We present a new functional method that is specifically designed to overcome these problems and include the external confining geometry exactly in the strongly interacting regime to linear order in the inverse interaction strength. Furthermore, it can be used to interpolate from few to mesoscopic particle numbers and address how spatial correlations emerge and evolve [13] , [14] , [15] , [16] . Our basic example below is a four-body system of two spin up and two spin down fermions in an external trap that is solved exactly for the first time here. Direct access to the wave function allows us to see ferro- and antiferromagnetic correlations in the eigenstates and give exact probabilities for these configurations. This is an extremely important feature of this new approach as multicomponent systems become highly degenerate for strong interactions, and thus the energy itself yields little information about the system. Furthermore, we solve exactly the impurity or polaron problem of one spin down interacting strongly with a number of spin up particles in a harmonic trap, a set-up that has been realized experimentally [16] . This allows us to compare different confining potentials and show that correlations are strongly influenced by the geometry. This has ramifications on density functional approaches for strong interactions, and our scheme can provide invaluable benchmarks of procedures where Bethe ansatz solutions obtained with periodic boundary conditions are supplemented by the local density approximation. For finite particle numbers, periodic boundary conditions is a strong assumption whose justification can now be addressed using exact solutions. Ultimately, our method could realize the goal of answering the key question: how many particles does it take to make a strongly interacting many-body system? Derivation of the energy functional The general system we consider has N particles of mass m with coordinates x 1 ,…, x N and is described by the Hamiltonian where p i is the momentum operator of particle i and V ( x i ) is an external confining potential. We assume a short-range two-body interaction that we model by a Dirac delta function of strength g . In the following, we are interested in the strongly interacting limit where g →∞ (or 1/ g →0). For simplicity, our focus will be the repulsive case ( g >0), although our results can be extended linearly to the attractive side ( g <0) of 1/ g =0. The deeply bound states for g → −∞ (refs 17 , 18 ) are irrelevant for our arguments and will not be addressed here. The external potential produces an energy scale, ε , and a length scale, l , in which we will express all other quantities. In the examples below, we will consider a double-well potential, V ( x )= mω 2 (| x |− b ) 2 /2, with barrier parameter, b , and a hard wall potential of length L that vanishes for 0< x < L and has infinite strength for x <0 and x > L . A double-well potential has recently been realized experimentally [15] , [19] . For b =0, the double well reduces to the harmonic oscillator potential from which we adopt our units of length, , and energy, ε = ℏ ω . Here ω is the oscillator angular frequency and ℏ = h /2 π is the reduced Planck’s constant. For the hard wall, we have l = L and ε = ℏ 2 /2 mL 2 . Henceforth, we will measure lengths, energies and g in these units. Our focus will be on fermions with two internal spin states, up and down. Systems with more than two internal states can be addressed in a similar manner (see Methods). A general eigenstate wave function has the form Ψ( x 1 ,…, x N ). For simplicity, we omit the coordinates from now on. The zero-range interaction implies that Ψ obeys the boundary conditions where the ±subscripts indicate the limits x i − x j →0 ± , that is, they are derivatives from each side of the point x i = x j . In the limit where 1/ g →0, the boundary conditions and the Pauli principle imply that Ψ must vanish whenever x i = x j for any i and j . Such functions can be constructed from the eigenstates of the single-particle Hamiltonian (the first term in equation (1)) by taking the antisymmetrized product of N states. This state we denote Ψ A . Its energy, E A , is a sum of the occupied single-particle energies. However, the boundary conditions allow us to write a more general state on the basis of Ψ A [9] , [20] , [21] , [22] , where we sum over the N ! permutations, P k , of the N coordinates, and θ ( x 1 ,…, x N )=1 when x 1 < x 2 <…< x N and zero otherwise. Fortunately, symmetries reduce the number of independent a k coefficients. For the present case of two-component fermions, the Pauli principle dictates that there are only M = N !/( N ↑ ! N ↓ !) degrees of freedom. This is the number of degenerate states at 1/ g =0, which shows that the functions in equation (3) constitute a basis. The basic idea is now very simple. To linear order in 1/ g we can write E = E A − K / g , where K = K ( a 1 ,…, a M ) is a functional of the a k coefficients and is independent of g by the Hellmann–Feynman theorem. One can now prove that K has the simple form (see Methods) where k and p run from 1 to M , and α k , p are matrix elements that depend only on the single-particle potential, V ( x ). The eigenfunctions and eigenenergies to order 1/ g can now be obtained by variation of K with respect to a k and diagonalizing the resulting matrix. K is equivalent to Tan’s contact parameter [23] in 1D [24] and we compute it exactly for 1/ g →0. Furthermore, the derivation can be easily extended to multicomponent bosons, fermions or mixtures, and it provides an effective Hamiltonian that can be used to study perturbations in the strongly interacting limit (see Methods for details). Remarkably, in the strongly interacting regime, the effective Hamiltonian can always be written as a spin model. In the important case of N spin 1/2 fermions or two-component bosons governed by the Hamiltonian in equation (1), it is a Heisenberg model of the form (ref. 25 , 26 ), which is a favourite starting point for research into quantum magnetism [27] . Here S i is the spin operator of particle i . It has been shown [20] that for a half-filled Hubbard model, J i = J is constant. This is obtained by using the Bethe ansatz and by the same method one can also prove that J i = J for particles in hard wall (box) confinement [28] . Our approach generalizes these important results and not only do we find that J i depends on the external confinement but also provide a procedure for computing these nearest-neighbour interaction coefficients exactly. We may therefore use the external confinement to tailor the J i coefficients into desirable spin models and thus manipulate static and dynamic quantum magnetic correlations [26] . Note also that this is not only true for the ground state manifold but also for higher manifolds as illustrated in Fig. 1a . Each manifold will have its own unique set of J i coefficients that we can compute exactly. In the language of the Hubbard model, one can think of higher manifolds as belonging to higher bands. 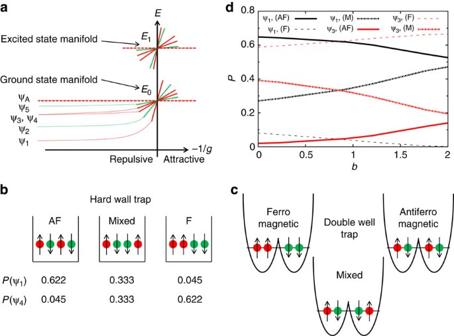Figure 1: Four-body system with two spin up and two spin down particles. (a) Schematic spectrum of eigenstates showing the ground state and an excited state manifold. The slopes at infinitegwill generally be different aroundE0andE1. For the ground state manifold, we indicate the adiabatic connection between the strongly and weakly interacting regime for a harmonic trap (b=0). The red lines are positive, while the green lines are negative parity states. The structure around 1/g=0 is the same for both double-well and hard wall traps, although the slopes are different. (b) Hard wall trap configurations and their probabilities for Ψ1and Ψ4that have opposite antiferromagnetic (AF) and ferromagnetic (F) contributions. The probabilities include both the configurations shown and their parity inverted partners that are equal. (c) Same asbfor the double-well trap. (d) The probability to find the three configurations incas function of the barrier parameter,b, for the ground state, Ψ1, and an excited state, Ψ3. Figure 1: Four-body system with two spin up and two spin down particles. ( a ) Schematic spectrum of eigenstates showing the ground state and an excited state manifold. The slopes at infinite g will generally be different around E 0 and E 1 . For the ground state manifold, we indicate the adiabatic connection between the strongly and weakly interacting regime for a harmonic trap ( b =0). The red lines are positive, while the green lines are negative parity states. The structure around 1/ g =0 is the same for both double-well and hard wall traps, although the slopes are different. ( b ) Hard wall trap configurations and their probabilities for Ψ 1 and Ψ 4 that have opposite antiferromagnetic (AF) and ferromagnetic (F) contributions. The probabilities include both the configurations shown and their parity inverted partners that are equal. ( c ) Same as b for the double-well trap. ( d ) The probability to find the three configurations in c as function of the barrier parameter, b , for the ground state, Ψ 1 , and an excited state, Ψ 3 . Full size image Four-body systems A central example is the hitherto unsolved four-body problem since it illustrates the method and it allows us to address magnetic correlation physics. We take N ↑ = N ↓ =2 with an M =4!/(2!) 2 =sixfold degeneracy at 1/ g =0 as shown in Fig. 1a for the case of a harmonic trap ( b =0). In general, the spectrum around 1/ g →0 has the form of a ladder of manifolds each of which contains an M -fold ‘fan’ of states as illustrated in Fig. 1a . For the ground state manifold we also show the adiabatic connection of states from weak to strong coupling where the third and fourth excited states are initially degenerate at g =0. The parity invariance of the double well and hard wall potentials means that the three types of spatially correlated states shown in Fig. 1b,c , ferromagnetic, antiferromagnetic and mixed, completely specify all solutions at 1/ g =0. Figure 1b shows the configuration probabilities for Ψ 1 and the state Ψ 4 for the hard wall, which turns out to have exact opposite ferro- and antiferromagnetic probabilities compared with the ground state. In Fig. 1d we show the double-well probabilities as functions of b for Ψ 1 and Ψ 3 , again picked as examples because of their significantly different correlations. In both cases we find a ground state that is dominantly spatially antiferromagnetic, and perhaps more remarkably we find excited states that are dominantly spatially ferromagnetic. Preparing different states at g =0 and then tuning to 1/ g =0 (refs 14 , 16 ) would thus produce completely different correlation patterns. Note that if one considers two-component bosons instead of fermions the results are very different (see Methods). One can understand intuitively what is going on by looking at equation (4). The antiferromagnetic configuration is favoured since ( a i − a j ) 2 is large for a i and a j differing in both sign and magnitude. The functional approach presented here thus provides a very precise mathematical insight into the preference for domain walls of opposite spin in the strongly interacting regime and provides a spatial explanation of antiferromagnetism in repulsively interacting 1D systems. Moreover, our results also demonstrate the potential for manipulating correlations by state preparation and trap shape modulation. A step in this direction was recently reported using anisotropic optical lattices [15] . Most often one discusses ferromagnetism induced by symmetry breaking. We clearly have the presence of a degenerate manifold of states to induce such breaking and a small spin gradient is enough to drive the system into a purely ferromagnetic state. However, our direct access to the exact wave function demonstrates the presence of intrinsic magnetic correlations even without breaking the spin symmetry. More generally, our method can be used to study the correlations that drive quantum phase transitions in larger systems using exact wave functions. Impurity problems As another demonstration of the nature of the strong coupling regime, we consider the case of a single spin down (impurity) interacting with a variable number of spin up fermions. An impressive recent experiment has considered this system for N ≤6 (ref. 16 ). As the energy at 1/ g →0 is degenerate, further insight into the strongly interacting regime has to come from correlations in the N -body wave functions. Here we consider the probability for the impurity to tunnel out of the trap as shown in Fig. 2a . In a simple model, we assume that because of the strong repulsion only the particle on the far right can tunnel out as the barrier is lowered (see Methods for details). Since the wave function in equation (3) contains a superposition of states with the impurity in different positions, the probability is simply given by the amplitude for it to be on the right, a N . In Fig. 2b we plot the impurity tunnelling probability, P ↓ =| a N | 2 , for N =2,…, 10 for the ground state of both a harmonic trap and a hard wall potential (see Methods for details). The results for N =2 and 3 are trap-independent, while for N ≥4 we see a clear geometrical dependence. In particular, we find that the scaling with N is completely different; whereas by a fit we find approximately P ↓ ∝ N −3 for the hard wall, the harmonic trap is not a power law but rather closer to a 1/ N ! behaviour as seen in the inset of Fig. 2b . The exact results thus allow us to conclude that geometry has a strong effect on correlations in the wave function. The exact wave functions also show that the impurity has a peak in its probability density at the centre of the trap. This is already true for N =3 and shows that for strongly interacting systems, studying the few-body limit gives insight into the behaviour of larger systems. Also note that the combination of McGuire’s solution (using periodic boundary conditions) [4] and the local density in the trap [29] can only capture the energy in the strongly interacting regime but does not reproduce the energy slope to order 1/ g . The 1/ N line in Fig. 1b applies to the non-interacting state Ψ A (which is often referred to as the 'fermionized' state). More importantly, 1/ N is also the probability obtained if the spin up particles had instead been strongly interacting bosons (see Methods for further details). This demonstrates a very strong deviation from the common perception of the similarity of strongly interacting fermions and bosons in 1D. 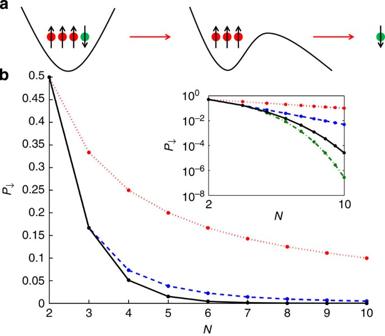Figure 2: Tunnelling of a strongly interacting impurity in a Fermi sea. (a) Illustration of a tunnelling experiment where the trap is opened on one side and the out-going particle and its spin is detected14for the case ofN↑=3 andN↓=1. (b) Probability to find the spin down impurity on the far right forN↑=1,⋯, 9 in ab=0 harmonic trap (solid) and a hard wall trap (dashed) for the ground state. The dotted line is 1/Nand is the probability in both traps for the non-interacting state, ΨA. It is also the result if theN↑majority particles are strongly interacting identical bosons. The inset shows the same data on a double-log plot. The dash-dotted line is 1/N! for comparison. Figure 2: Tunnelling of a strongly interacting impurity in a Fermi sea. ( a ) Illustration of a tunnelling experiment where the trap is opened on one side and the out-going particle and its spin is detected [14] for the case of N ↑ =3 and N ↓ =1. ( b ) Probability to find the spin down impurity on the far right for N ↑ =1, ⋯ , 9 in a b =0 harmonic trap (solid) and a hard wall trap (dashed) for the ground state. The dotted line is 1/ N and is the probability in both traps for the non-interacting state, Ψ A . It is also the result if the N ↑ majority particles are strongly interacting identical bosons. The inset shows the same data on a double-log plot. The dash-dotted line is 1/ N ! for comparison. Full size image The strongly interacting regime is very difficult to access both numerically and analytically because of many (nearly) degenerate energy eigenstates. The present approach finds the exact solution to linear order in 1/ g in a manner that automatically yields eigenstates that are adiabatically connected to the eigenstates for smaller values of g . Combining our analytical approach with numerical techniques that perform well in the weakly and intermediate strength regime will allow us to access the quantitative and qualitative behaviour of 1D systems in arbitrary confining geometries. Furthermore, our approach provides a necessary starting point for including higher orders in 1/ g (refs 30 , 31 ) and it represents an essential benchmark for numerical calculations. [17] , [18] , [25] contain recent numerical calculations very close to the 1/ g =0 limit. The results presented here are in agreement with those calculations. A leading numerical method used for 1D systems is the density matrix renormalization group technique. As this is intrinsically a variational approach, it is not clear how well it will perform in strongly interacting limit for multicomponent systems where the degeneracy of the spectrum is large. In addition, our method can provide a fairly simple benchmark of density matrix renormalization group by using the exact slopes of the energy as 1/ g →0. It is extremely important to note that with no extra effort our method obeys the Lieb–Mattis theorem [32] , which states that the energies may be ordered according to total spin, S , with the ground state having the minimal S . It is tempting to conclude that the exact solution can be obtained by constructing eigenstates with well-defined total spin at 1/ g =0, and many previous attempts to solve this problem have been based on spin algebra and spin mappings in one way or another [21] , [22] . However, this construction is not unique and our method demonstrates that the condition is insufficient to determine the eigenstates to order 1/ g for N >3 for multicomponent systems where M >3. Insisting on states that are eigenstates of the total spin provides just one extra constraint and this is not enough to determine all the coefficients a k . A more direct way to see that the spin algebra approach is incomplete is to note that the construction of the spin functions ignores the confinement V ( x ) [22] . While it does yield eigenstates in the strict limit 1/ g =0, the spin states obtained for N >3 are generally not adiabatically connected to states at large but finite g . The method presented here overcomes this naturally by extremizing the slope of the energy as the criteria that determines the eigenstates. Several previous papers have introduced Bose–Fermi and Fermi–Fermi duality mappings for interacting 1D systems [33] , [34] , [35] , [36] . This is a very nice mathematical tool for transforming between strongly and weakly interacting systems; however, it must be stressed that these techniques cannot be used to solve the problem considered here. Many of these techniques start from the antisymmetrized noninteracting state and then multiplies by a factor that ensures that under exchange of two particles the sign comes out correctly (plus for two bosons and minus for two fermions). As we have clearly shown, the coefficients ( a k ) are generally not integer. For multicomponent systems and for Bose–Fermi mixtures, duality mappings must be supplemented by knowledge of the solution on either the fermion or boson side of the duality transformation. Without our solution one would merely be mapping into another unsolved problem. On the other hand, combining our technique and duality transformations we expand the class of solvable systems. Details of the energy-functional derivation As noted in the main text, in the strongly interacting limit, 1/ g →0, the boundary conditions in equation (2) imply that the total wave function Ψ must vanish whenever x i = x j . For two identical fermions, this is trivial since the Pauli principle dictates that both sides of equation (2) vanish. For non-identical particles, the wave function must still vanish when they overlap; however, the derivatives from each side can generally be different since the Pauli principle provides no restrictions. The basic idea of our method is now very simple. First construct an antisymmetric function, Ψ A , with energy E A using single-particle states as described in the main text. The most general N -body wave function is shown in equation (3). The number of independent coefficients in equation (3) can be deduced from Pauli symmetry to be M = N !/ S , where the symmetry factor is calculated according to the number of groups of identical particles in the system; S = N 1 ! N 2 !… N n ! if there are n groups of identical particles with N 1 , N 2 ,…, N n in each group. Now we can construct an energy-functional, K ( a 1 ,…, a M ), such that E = E A − K / g . Subsequently, we vary K with respect to a k and diagonalize the resulting linear system to obtain the exact eigenstates and slopes of the energy to linear order in 1/ g . Intuitively, the functional gives the slopes of the energy so that the ground state on the repulsive side ( g >0) around 1/ g =0 will maximize K , the first excited state will be the next extreme point, and so on. The proof of equation (4) is an exercise in application of techniques from standard quantum mechanics. Using either perturbation theory or the Hellmann–Feynman theorem, we have where the Dirac bracket ‹Ψ|Ψ› denotes the normalization integral. The dependence on g can be eliminated by using equation (2) in equation (5) that yields where it is important that one first evaluates the derivatives and then integrates out the delta function. Note that if i and j are the indices of identical fermions, then the Pauli principle requires antisymmetry under permutation and we get a vanishing contribution to K . We can now split this integral into N ! sectors with different particle orderings, that is, where we sum over permutation of the coordinates, P k , and the integration regions, Γ k , are such that . This is very much in the spirit of the Bethe ansatz of course. In the Bethe ansatz, the assumption is that the two-body potential scatters without diffraction [37] . In our case, the very notion of scattering is compromised by the presence of the external trap and not even asymptotically can we talk about free particles in a general confining 1D geometry. Here we use instead the local properties of the two-body interaction. From every boundary where two particles coincide, we will obtain a factor ( a k − a p ) 2 times a derivative of Ψ A . If they are identical fermions, then a k = a p and the term vanishes; however, to keep it general we do not make such an assumption here. K can thus be written as a sum of quadratic differences of the a k coefficients. Likewise, we may use the normalization (corresponding to unit normalization on each of the M sectors in the expansion equation (3)). Therefore, K can be written as where k and p run over the number of independent coefficients M = N !/ S and we have used the antisymmetry of Ψ A to eliminate the factor 1/4. This is equation (4) of the main text. The quantity α k , p is defined as In addition, we first have to take the derivative before integrating over the delta function. Here P k is a permutation of the coordinates that has the property that x i and x j are next to each other so that they can interact, while p denotes a permutation, P p , of the same kind but with x i and x j in reverse orders. This shows why we do not need to put the index p explicitly on the right-hand side since it is uniquely specified for given k , i and j . Note that these integrals will generally also depend on the ordering of all the other particles besides x i and x j , which is specified by P k . The decisive observation is that the ground state in the vicinity of 1/ g →0 will be the state that maximizes the slope K . In fact, all sets of a k that extremize K define a wave function that is an eigenstate around 1/ g →0, and these will be orthogonal. This is proved as follows. First define a basis of states given by setting a k =1 and a p =0 for p ≠ k ; this defines a set of M so-called bump functions that all have energy E A through Ψ A . We now apply degenerate perturbation theory to first order, which yields a secular matrix (to be discussed below) whose eigenvalues are the slopes K i and eigenstates are the correct eigenfunctions for 1/ g →0. The result now follows from the linear variation method, which states that the extremizing combinations are orthogonal eigenstates. We have just shown that we can use either degenerate perturbation or variation to find the exact wave functions for the ground state for 1/ g →0 and we obtain the slopes, K , automatically. It is straightforward to argue for the adiabatic connection of the ground state at g =0 and the ground state around 1/ g →0 + for the lowest E A value possible where Ψ A constructed by one particle in each of the N lowest single-particle states. This follows from the Lieb–Mattis theorem and the fact that the largest total spin state is uniquely defined. For higher states, one must be more careful in connecting the states, and symmetry classifications at both weak and strong interactions is a very useful tool [38] . However, we stress that symmetries (permutation group, parity invariance and so on) cannot be used to determine the a k coefficients themselves for general external confinement and arbitrary number of particles. The determination of the amplitudes, a k , now proceeds by linearization of the functional, ∂ K /∂ a k =0. This produces an eigenvalue equation of the form A υ= K υ, where υ is a vector with a k as entries, while A is a symmetric matrix containing combinations of the α k , p coefficients. By diagonalizing A we obtain the orthogonal and complete set of eigenstates. This completes the proof of the solvability of the strongly interacting problem in an arbitrary confining potential in 1D to linear order in 1/ g . The derivation above allows us to write down the effective strong interaction Hamiltonian H eff = E A I M −(1/ g ) A , where I M is an M -dimensional identity matrix. H eff can be used to study additional perturbations on the system such as external electromagnetic fields in the strongly interacting regime. The exact solutions generically have different a k coefficients (in fact a subset of coefficients can even vanish in a given eigenstate). This explains why it is very difficult to achieve convergent results in the strongly interacting limit using numerical techniques that are not optimized to take this into account. By taking different Ψ A with different energies E A we can now build the entire spectrum that will consist of a ladder of states each with an M -fold degeneracy at 1/ g =0 and determine their slopes, K , around 1/ g =0. This is illustrated for ground state and excited state manifolds in Fig. 1 in the main text. Fermions with I >2 internal states or colours (such as an SU ( I ) model) are solved by exactly the same method but with a different M , depending on the number of such colours. A minor adjustment for strongly interacting bosons is that when two identical bosons are interchanged in permutations P k and P p of equation (4), we must take a k =− a p to compensate the antisymmetry of Ψ A and consequently add a term to the numerator in equation (8) to account for the interactions in equation (1). Mixtures of fermions and bosons run along the same lines. Our only assumptions are that the particles have equal masses, the same interaction strength g between all components and a confining potential, V ( x ), which is the same for all particles. Details for four-body systems The two spin up and two spin down systems discussed in the text have the general wave function where we have fixed x 1 and x 2 to be spin projection up, while x 3 and x 4 have spin projection down. The topology of each configuration is indicated by the arrows. Note that we have only written the independent pieces of the wave function; the remaining terms are dictated by the Pauli principle. In the example we consider the ground state manifold (lowest energy at 1/ g =0), meaning that Ψ A ( x 1 , x 2 , x 3 , x 4 ) is the antisymmetric function formed by occupying the four lowest states in the confining potential. The functional for the energy around 1/ g =0 using this basis becomes where we notice the absence of a term with α 3,4 since those configurations have no matching boundaries. By using parity invariance, one sees that α 1,2 = α 5,6 ≡ α and α 2,3 = α 2,4 = α 3,5 = α 4,5 ≡ β , so that we have only two independent coefficients. By variation of K with respect to a k , we obtain the A matrix that has the rather simple form and acts on the vector υ=[ a 1 , a 2 , a 3 , a 4 , a 5 , a 6 ] T , where the superscript T denotes the transpose. Note how parity symmetry is explicitly featured in A since it is symmetric when reading it from the top left corner to the bottom right corner or vice versa . The explicit forms of α and β are where the difference between the two quantities is the ordering of coordinates in the integration region. Integrating out the delta function and renaming the variables in α ( x 4 → x 3 ) show that we have x 1 < x 2 < x 3 and x 1 < x 3 < x 2 , respectively. An easy way to think about the difference is that β has the pair that interacts on the side of the system (left and right sides are equivalent because of parity invariance), while for α the interacting pair is in the middle. These two are generally not the same. However, for the particular case of the hard wall confinement, it turns out that α = β . In this case our results are consistent with the Bethe ansatz approach [28] . For the double-well potential, α ≠ β . This is perhaps a subtle point even to experts in the field and may explain a number of previous failed attempts to obtain the exact solution. By diagonalization of A we obtain the slopes and wave functions that allows us to determine the structures and probabilites discussed in the main text. For the case where the two pairs of identical particles are instead bosons, there are additional interaction terms when the two identical bosons are next to each other. The modification to the A matrix is very simple and consists of adding a diagonal matrix diag(4 β , 0, 2 α , 2 α , 0, 4 β ) to A . The ground state is then of the simple form υ=[1,−1,1,1,−1,1] T , which is easily seen to correspond to Ψ=|Ψ F | where Ψ F is the wave function for spinless fermions, that is, the Girardeau wave function [9] . Thus, we get uniform probability of 1/3 for each of the three configurations shown in Fig. 1 . In addition, we notice the differences between strongly interacting bosons and fermions. Details for polaron systems The fermionic polaron system where a single spin down (often called an impurity for obvious reasons) interacts with a number of identical spin up fermions is handled in a similar manner to the four-body system, although the A matrix has an even simpler structure. Let the single spin down particle have coordinate x 1 , and the N −1 spin up particles have coordinates x 2 ,…, x N . There are N !/( N −1)!= N independent a k coeffiecients. The wave function is now given by It is now straightforward to obtain the slope, which is given by As before, we can use parity invariance of the confinement to conclude that α 1,2 = α N −1, N , α 2,3 = α N −2, N −1 and so forth. This means that the number of independent α i , j is N /2 for N even and ( N −1)/2 for N odd. The corresponding A matrix is tridiagonal with entries The different coefficients of the matrix are for k =1,…, N /2 for N even and k =1,…, ( N −1)/2 for N odd. Here the integral is over the region Γ= x 2 < x 3 <…< x 1 < x k +1 <…< x N . In addition, we note that these constants are not equal for general potentials. However, once more the hard wall confinement is a truly special case. There one can prove that the α k , k +1 are equal and one recovers the Bethe ansatz results [28] . The results above can be applied to the case where x 2 ,…, x N are identical bosons instead of fermions. For the Hamiltonian in equation (1) with a single coupling, g , for all pair-wise interactions, the ground state is the one found by Girardeau many years ago [9] since the Hamiltonian does not distinguish between the identical bosons and the impurity. Alternatively, by counting interacting pairs in each configuration one can show that in a hard wall confinement the two-component boson case is obtained by adding a diagonal matrix to A of the form diag(2( N −2), 2( N −3), 2( N −3),…, 2( N −3), 2( N −2)). Note that the inter- and intraspecies interactions are the same for these two-component bosons, and the coupling constant goes to infinity (1/ g →0). This follows from the structure of our Hamiltonian that does not distinguish between the two species. An interesting example of non-identical inter- and intraspecies interactions can be found in ref. 39 . For general potentials with nonconstant α k , k +1 , the matrix to add will still be diagonal but now the entries are sums over a set of α k , k +1 with a contribution from each adjacent pairs of identical bosons for a given configuration. Let us denote the two species as A and B and consider the example with three A -type bosons and one B -type (acting as the impurity). In this case the four diagonal terms (corresponding to configurations BAAA , ABAA , AABA and AAAB ) are 2( α 2,3 + α 3,4 ) for BAAA and also for AAAB , and 2 α 1,2 for ABAA and also for AABA (there is symmetry around the centre of the diagonal because of the parity symmetry of the potential). Thus, in the limit | g |→∞, we have the ground state wave function Ψ=|Ψ A |. This has probability 1/ N for the impurity to sit on the right-hand side of the system. This is a clear demonstration of the differences between fermions and bosons when there are multiple internal states. Our formalism can also be applied to a mixture with N 1 single component fermions and N 2 single component bosons. However, if the Bose–Fermi and Bose–Bose zero-range interactions have different strength parameters, then the situation changes drastically and the ground state depends on the ratio of these strength parameters as they diverge to infinity [39] . Tunnelling The tunnelling problem considered in the main text is considered within a simple model that can be justified in several different ways. Here we will use arguments based on the many-body tunnelling theory of Bardeen [40] . It has recently been shown [41] that the Bardeen theory can reproduce experimental results on strongly interacting two-body systems [14] , and we assume that this remains true for more particles as studied in the main text. We assume that the exact eigenstate we have obtained is the initially stationary state that starts to decay as the barrier is lowered. This initial state can be written as a sum of eigenstates of the new Hamiltonian with a lowered barrier, and we arrive at a dynamical problem. While this may sound very complicated, the new Hamiltonian is still assumed to be strongly interacting and particles are still not allowed to exchange positions. The particle that was initially closest to the barrier before it is lowered will therefore provide the dominant contribution to the flux going out of the trap. The initial state therefore contains the information about the tunnelling rates. This can be made quantitative by computing very accurate matrix elements for the rates. Since our main purpose is to point out the difference of different initial states in tunnelling experiments, we postpone further tunnelling calculations for future studies. How to cite this article : Volosniev A. G. et al. Strongly interacting confined quantum systems in one dimension. Nat. Commun. 5:5300 doi: 10.1038/ncomms6300 (2014).